Anisotropic thermal conductivity in uranium dioxide The thermal conductivity of uranium dioxide has been studied for over half a century, as uranium dioxide is the fuel used in a majority of operating nuclear reactors and thermal conductivity controls the conversion of heat produced by fission events to electricity. Because uranium dioxide is a cubic compound and thermal conductivity is a second-rank tensor, it has always been assumed to be isotropic. We report thermal conductivity measurements on oriented uranium dioxide single crystals that show anisotropy from 4 K to above 300 K. Our results indicate that phonon-spin scattering is important for understanding the general thermal conductivity behaviour, and also explains the anisotropy by coupling to the applied temperature gradient and breaking cubic symmetry. Today nearly 20% of the world’s electricity is generated by nuclear energy from UO 2 fuel. The thermal conductivity of UO 2 governs the conversion of heat produced from fission events into electricity and it is an important parameter in reactor design and safety. Scatter among thermal conductivity ( κ ) data from previous experimental studies on UO 2 single crystals cannot easily be explained by sample impurities or inherent measurement errors. (see ref. 1 and references therein). We hypothesize that much of this scatter is due to hidden anisotropy, overlooked in previous experiments that did not specify single crystal orientation. The crystal symmetry of materials dictates the symmetry of the response to applied potential gradients. Thermal conductivity is a second-rank tensor (that is, κ = κ ij ) that governs the flow of energy under an applied temperature gradient. For materials with cubic point and space group symmetry it is isotropic. Thermal conductivity is almost exclusively dominated by phonons in insulators and semiconductors. At very low temperatures, where ballistic phonon transport may occur, exceptions to the isotropy of cubic materials have been reported, for example, ref. 2 . This can be explained by the thermal conductivity being a fourth rank tensor ( κ = κ ijlm ) related to the elastic stiffness tensor when phonon scattering is minimal [3] . Here we show by experiments on single crystals that UO 2 , which crystallizes in the cubic fluorite structure , exhibits anisotropic thermal conductivity at temperatures at which ballistic mechanisms are not possible. The anisotropy is rather due to the applied temperature gradient interacting with the electric moments on uranium ions thus affecting the phonon-spin interactions to slightly break cubic symmetry. This effect is caused by the magnetic properties of UO 2 and the degenerate bands giving rise to Jahn–Teller distortions. This result is unexpected since the crystal structure for both the paramagnetic and the antiferromagnetic phases of UO 2 are cubic and there is no clear evidence of non-cubic distortions in diffraction experiments [4] . These results should also apply to the interpretation of other magnetic strongly correlated materials exhibiting Jahn–Teller physics [5] . Molecular dynamics simulations of UO 2 thermal conductivity Our consideration of anisotropic UO 2 thermal conductivity originated from molecular dynamics (MD) simulations using the direct method [6] , [7] , [8] , which calculates thermal conductivity by measuring the temperature gradient in a rectangular cuboid with heat added and removed at a hot and cold plate, respectively. The simulations predict large differences for the effective thermal conductivity in the <100> <110> and <111> crystallographic directions at 300 K, see Fig. 1a . In an attempt to eliminate boundary condition artifacts related to scattering by the hot and cold plates, the thermal conductivity is obtained for infinite simulation cell length by extrapolation [7] , [8] . 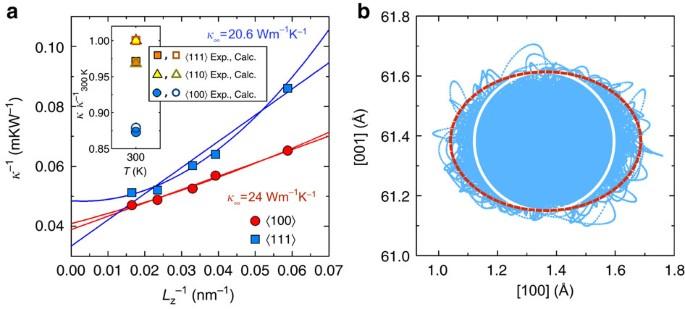Figure 1: Anisotropic UO2thermal conductivity from MD simulations. (a) The thermal conductivity (κ) variation (κ−1) as a function of the lengthof the simulation cell for the temperature gradient applied in the <100> and <111> lattice directions at 300 K. The lines represent linear and quadratic fits to the data used for extrapolation to infinite length (κ∞) of the simulation cells7,8. The inset compares the experimentally measured thermal conductivity values (Exp.) in the <100> <110> and <111> crystallographic directions with the MD simulations (Calc.). The length of the MD simulation cells were ~30 nm for these data points. The values have been normalized to the highest thermal conductivity value at 300 K (κ300). (b) Projected trajectory of one oxygen ion during a 500 ps MD run in the rectangular cuboid simulation cell at 300 K. The MD simulation was performed in the NVE ensemble without an applied thermal gradient. The horizontal axis is the [100] and the vertical axis the [001] direction of the fluorite lattice. The elongated direction of the simulation cell is along the vertical axis. The ellipsoid character of the distribution is emphasized by the dashed red line as compared with the white line representing the spherical distribution. Figure 1a shows that ( L z is the length of the simulation cell) does not obey the expected linear relationship for UO 2 in the <100> direction, and is instead quadratic. The extrapolated values at 300 K in the inset of Fig. 1a (based on the quadratic fits) show that the anisotropy between <111> and <100> is ~15%. This result is noteworthy as the quadratic term indicates that the intrinsic material properties are affected, whereas a linear term would correspond to a mere change in the phonon scattering length. The underlying physics is illustrated by the projected MD trajectory of an oxygen ion, see Fig. 1b . This simulation was performed in the same rectangular cuboid cell as the thermal conductivity simulations, but without a temperature gradient. Although the average position coincides with the cubic UO 2 fluorite structure, the shape of the distribution is an ellipsoid rather than the expected sphere. The ellipsoidal character is still present during short time intervals in a cubic simulation cell, however it averages to a sphere since the ellipsoid orientation along the crystallographic axes is uncorrelated in space and time. Apparently, the trajectory is sensitive to small perturbations, such as the dimensionality of the simulation cell or the applied temperature gradient. These perturbations break the underlying cubic symmetry, and lead to a preferential ellipsoid orientation along one of the three <100> axes. This orientation bias gives rise to anisotropy in the physical properties. Figure 1: Anisotropic UO 2 thermal conductivity from MD simulations. ( a ) The thermal conductivity ( κ ) variation ( κ −1 ) as a function of the length of the simulation cell for the temperature gradient applied in the <100> and <111> lattice directions at 300 K. The lines represent linear and quadratic fits to the data used for extrapolation to infinite length ( κ ∞ ) of the simulation cells [7] , [8] . The inset compares the experimentally measured thermal conductivity values (Exp.) in the <100> <110> and <111> crystallographic directions with the MD simulations (Calc.). The length of the MD simulation cells were ~30 nm for these data points. The values have been normalized to the highest thermal conductivity value at 300 K ( κ 300 ). ( b ) Projected trajectory of one oxygen ion during a 500 ps MD run in the rectangular cuboid simulation cell at 300 K. The MD simulation was performed in the NVE ensemble without an applied thermal gradient. The horizontal axis is the [100] and the vertical axis the [001] direction of the fluorite lattice. The elongated direction of the simulation cell is along the vertical axis. The ellipsoid character of the distribution is emphasized by the dashed red line as compared with the white line representing the spherical distribution. Full size image Measurements of anisotropic UO 2 thermal conductivity These MD results inspired a detailed experimental study of the UO 2 thermal conductivity as a function of temperature with a thermal gradient applied in different crystallographic directions on oriented single crystal bars. We find that the overall shape of the thermal conductivity is atypical for insulating crystals without defects, see Fig. 2 . For all directions, pronounced double-peak behaviour in the thermal conductivity is observed with maxima occurring at ~10 and 220 K and a minimum at the Néel temperature T N =30.8 K, as reported previously [1] , [9] . This behaviour has been observed in other materials with antiferromagnetic transitions [9] , [10] , [11] , [12] , [13] , which is due to resonant scattering of phonons through excitations of the spins on the magnetic ions in the paramagnetic phase and absence of this scattering mechanism below T N due to spin ordering [9] , [10] , [11] , [12] , [13] . The temperature dependence of the UO 2 thermal conductivity below 10 K obeys κ ∝ T 1.45 , see Fig. 2b , which deviates from the expected κ ∝ T 3 dependence for phonons. Therefore we speculate that the low temperature UO 2 thermal conductivity is mediated by magnons, or magnons and phonons. 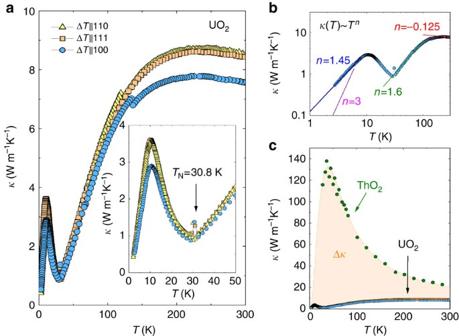Figure 2: Measured UO2thermal conductivity. (a) UO2thermal conductivity (κ) in the <100> <110> and <111> crystallographic directions (please refer to Methods for details on sample preparation and the thermal conductivity measurements). The inset highlights the thermal conductivity in the region of the Néel temperature (TN). The spike atTNis a consequence of the divergence of the heat capacity. (b) Log–log plot of thermal conductivity as function of temperature (T). (c) Measured UO2thermal conductivity compared with reference data for ThO2(ref.14). Figure 2: Measured UO 2 thermal conductivity. ( a ) UO 2 thermal conductivity ( κ ) in the <100> <110> and <111> crystallographic directions (please refer to Methods for details on sample preparation and the thermal conductivity measurements). The inset highlights the thermal conductivity in the region of the Néel temperature ( T N ). The spike at T N is a consequence of the divergence of the heat capacity. ( b ) Log–log plot of thermal conductivity as function of temperature ( T ). ( c ) Measured UO 2 thermal conductivity compared with reference data for ThO 2 (ref. 14 ). Full size image Regardless of the thermal transport mechanism below T N , scattering by spin excitations on the uranium ions are responsible for the unusual shape above this temperature [9] , see Fig. 2a . In particular: the maximum thermal conductivity is of low magnitude (8.7 W m −1 K −1 ), occurs at high temperature (220 K) and then decreases slowly. Typically the phonon thermal conductivity rises quickly and reaches its maximum well below 100 K, after which phonon–phonon scattering leads to rapid decrease. In UO 2 , scattering by the spins on uranium ions results in a lower thermal conductivity and higher temperature for the maximum conductivity than if only phonon–phonon scattering were active. This effect is illustrated in Fig. 2c , which compares the UO 2 thermal conductivity to recent measurements on ThO 2 single crystals [14] . ThO 2 is isostructural with UO 2 although it is diamagnetic [15] and thus there is no phonon-spin scattering. The maximum ThO 2 thermal conductivity is 140 W m −1 K −1 at about 40 K [14] , which is a more typical case for metal oxides. Scattering between phonons and spins on uranium ions occurs by phonons exciting the energy levels of the magnetic ions [10] , [11] , [12] , [16] , [17] , [18] . The magnitude of this resonant phonon-spin scattering mechanism is controlled by the position of these energy levels. Scattering is prominent if the excited spin states are in the same energy range as the occupied phonons, otherwise scattering is negligible [10] , [16] , [17] , [18] . There are no excitation levels in the triplet ground state of uranium ions above T N that can interact with phonons [19] , [20] . However, inelastic neutron scattering experiments have identified a dynamic Jahn–Teller distortion in <100> lattice directions that splits the ground state into three singlets with dispersive peaks of magnetic character between 3 and 10 meV [19] , [20] . These excitations are in the appropriate energy range for interaction with phonons and give rise to significant scattering in the paramagnetic phase. Analysis of UO 2 thermal conductivity We can gain further insight by analyzing the temperature dependence of the UO 2 thermal conductivity, which above T N can be represented by an extended Callaway model [21] (see Methods). This approach applies a Debye model for the phonon spectrum and considers scattering by boundaries, point defects and Umklapp phonon–phonon processes. A Callaway model for ThO 2 was modified to capture the important differences with UO 2 . This extension required a model for resonance spin scattering at two different energy levels ( , where τ S is the spin scattering relaxation time, ω is the phonon frequency, ω S is the resonance frequency, C is the phonon-spin coupling constant and F ( T ) describes the properties of the two-level system) [22] . In addition to the resonance terms, the defect scattering in UO 2 is increased compared with ThO 2 possibly due to isotopic contributions. These fits reproduce the UO 2 thermal conductivity data, see Fig. 3 . The resonance energy obtained for the <110> UO 2 data is about 3 meV (the two levels in the model overlap), which agrees with the lowest energy excitation measured in the inelastic neutron scattering experiments [19] , [20] . This result gives us confidence that the low UO 2 thermal conductivity and its unique temperature dependence are due to resonance scattering of phonons by excitations involving spins on the uranium ions. The Callaway model parameters are found in Supplementary Table 1 . 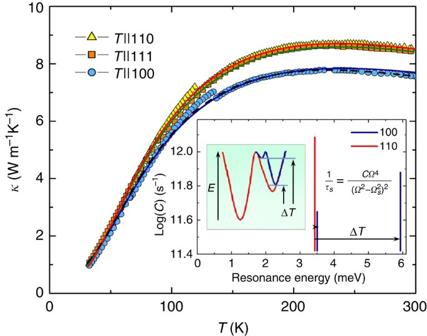Figure 3: Measured UO2thermal conductivity fitted to the extended Callaway model. Markers show the measured thermal conductivity (κ) data and lines the Callaway fits. The anisotropy is captured by shifting the energies (ħωS, whereħis the reduced Planck constant andωSis the resonance frequency) and coupling constants (C) in the resonance spin scattering terms, see equation in the inset. The difference in resonance scattering parameters for the <110> and <100> crystallographic directions is illustrated in the inset. The arrows show the shifts occurring due to the applied temperature gradient (ΔT) in the <100> direction. The second inset schematically illustrates the same shift and splitting in terms of potential wells (E). The dashed line for UO2<100> represents a fit where both the spin and Umklapp scattering terms were allowed to change, which differs from solid line where only the spin scattering terms were treated as free parameters. Figure 3: Measured UO 2 thermal conductivity fitted to the extended Callaway model. Markers show the measured thermal conductivity ( κ ) data and lines the Callaway fits. The anisotropy is captured by shifting the energies ( ħω S , where ħ is the reduced Planck constant and ω S is the resonance frequency) and coupling constants ( C ) in the resonance spin scattering terms , see equation in the inset. The difference in resonance scattering parameters for the <110> and <100> crystallographic directions is illustrated in the inset. The arrows show the shifts occurring due to the applied temperature gradient (Δ T ) in the <100> direction. The second inset schematically illustrates the same shift and splitting in terms of potential wells ( E ). The dashed line for UO 2 <100> represents a fit where both the spin and Umklapp scattering terms were allowed to change, which differs from solid line where only the spin scattering terms were treated as free parameters. Full size image At low temperature, anisotropic thermal conductivity in cubic materials has been previously observed and attributed to ballistic phonon transport or phonon focusing mechanisms [2] . However, these explanations are not possible in UO 2 because the short mean free path due to spin scattering rules out boundary scattering from macroscopic sample surfaces as the mechanism limiting phonon lifetimes. This conclusion is also supported by the anisotropy persisting at least 150 K above the maximum thermal conductivity. Sample impurities and oxygen non-stoichiometry were also ruled out as explanation for the anisotropy (see Methods). In addition, scattering due to the presence of different isotopes, which has important effect on other fluorite oxides (for example, CeO 2 , HfO 2 and ZrO 2 ), is not a significant issue in depleted uranium samples considered in this study (see Methods). ThO 2 has only one naturally occurring isotope and thus behaves similar to UO 2 with regards to isotope effects on thermal conductivity. Anisotropy of UO 2 thermal conductivity below T N Below T N the anisotropy may not seem surprising, since Jahn–Teller distortions of the oxygen sublattice exist [23] , [24] . This reduced symmetry originates from the transverse 3 k dipolar ordering and leads to a different space group: to (ref. 25 ). This behaviour is driven by similar ordering of the uranium electric quadrupoles [26] . While, has reduced symmetry with respect to it is still a cubic space group that requires that the thermal conductivity must fulfil cubic symmetry relations and cannot explain the anisotropy. Whether the thermal conductivity below T N is due to phonons, magnons or both, we suggest that the key to understanding the anisotropy is the [ ξ 00] optical magnon branches, and for phonon mechanisms, the scattering that they give rise to. Measurements of the magnon dispersion in UO 2 have revealed an optical [ ξ 00] branch with a minimum at the [100] reciprocal lattice point of around 2 meV (23.2 K) and a maximum at [000] of 10–12 meV (116.2–139.3 K) (refs 19 , 20 ), which is the required energy range to couple with phonons below T N . The [ ξ 00] magnons or the phonon–magnon scattering by themselves do not explain the observed anisotropy, since the cubic crystal symmetry dictates equal contribution from all [ ξ 00] branches. However, the temperature gradient applied during the thermal conductivity measurements interacts with the magneto-vibrational properties of the UO 2 lattice such that the [ ξ 00] branches are affected differently when the gradient is applied in, for example, the <100> <110> and <111> crystallographic directions. The temperature gradient alone does not give rise to this behaviour, but instead we propose that the small electric field generated by the temperature gradient is the source. This behaviour is facilitated by UO 2 having a large Seebeck coefficient [27] . We suggest that this field interacts with the electric moments on uranium ions in UO 2 to change the [ ξ 00] magnon properties. The fact that the major anisotropy occurs in the <100> direction coincides with the small C 44 elastic constant of UO 2 , the minimum of which is at T N (ref. 28 ). Anisotropy of UO 2 thermal conductivity above T N Above T N , the anisotropy is even more unexpected, since paramagnetic UO 2 has always been measured to be a perfect cubic fluorite. In this temperature range phonons in the paramagnetic phase are scattered by the resonant states that originate from splitting of the triplet ground state of uranium ions into singlets by the dynamical Jahn–Teller distortions [19] . These lattice distortions alone do not explain the anisotropy. As for below T N , we speculate that it is caused by the applied temperature gradient interacting with the magneto-vibrational properties and giving rise to different response when applied in the <100> <110> and <111> crystallographic directions. This can be viewed as the gradient slightly changing the character of the distortions. This mechanism was investigated by fitting the extended Callaway model to the <100> <110> and <111> experimental thermal conductivity results. The <110> model was used as a baseline and the other conductivities were then fitted by allowing the resonance scattering terms to change (see Methods). All other parameters were held fixed. The results shown in Fig. 3 reveal that the anisotropy in the <111> and <100> directions is accommodated by splitting and shifting the two resonance energies by 0.37 to 2.4 meV, and modifying the phonon-spin coupling constants. This situation is similar to reducing the symmetry by application of an external field [29] ; however, it is surprising that the small temperature gradients used in the thermal conductivity experiments have such a profound effect on the conductivity. An important feature of this model is that it explains the anisotropy of the thermal conductivity, while not requiring deviation from the cubic crystal structure measured in diffraction [4] . These findings are a result of the anisotropy arising from scattering processes that only develop non-cubic character in the presence of temperature gradients. The measured thermal conductivity values in the <111> and <110> directions agree with recent phonon lifetime measurements (8.4±1.5 W m −1 K −1 at 295 K compared with our measurements of 8.53 and 8.44 W m −1 K −1 for the <110> and <111> directions, respectively) [30] . Since lifetime measurements do not apply temperature gradients, it follows that the best agreement occurs for the <111> and <110> directions. These two directions do not couple to the applied temperature gradient, in contrast to the <100> direction for which the corresponding thermal conductivity is 7.59 W m −1 K −1 . The Callaway model for the different crystallographic directions can be used to extrapolate the thermal conductivities, which shows that the anisotropy remains even at high temperature, for example, it is predicted to be ~10% at 1,200 K. The small discontinuity in the thermal conductivity between 100 and 150 K coincides with the onset of anisotropy. The source of the discontinuity is still under investigation. Returning to the MD simulations, the phonon-spin scattering origin of the anisotropy cannot be captured since the empirical potential does not account for magnetism. Furthermore, the lack of explicit phonon-spin scattering models results in an overestimation of thermal conductivity compared with experiments, see Figs 1 and 2 . At 300 K, the simulated thermal conductivity values for UO 2 are closer to the experimental results for ThO 2 (no phonon-spin scattering) than to the UO 2 data. Nevertheless the fact that the empirical potential still captures the anisotropic response of UO 2 in a temperature gradient (see inset of Fig. 1a ), suggests that some of the physics arising from the phonon-spin scattering has been embedded into the force field description via the soft C 44 elastic constant and lattice anharmonicity [31] . In summary, the results of this study show that an applied temperature gradient interacts with the electric moments on uranium ions to slightly break cubic symmetry and leads to anisotropy in physical properties. Specifically, the measured and calculated anisotropic UO 2 thermal conductivity give clear evidence of UO 2 exhibiting properties of a non-cubic compound, because second-rank tensors, such as thermal conductivity, must result in isotropic behaviour for cubic materials. This result is unexpected since the crystal structure for the paramagnetic as well as the antiferromagnetic phases of UO 2 are cubic and there is no clear evidence of non-cubic distortions in diffraction experiments. MD simulations MD simulations applying the direct method [6] , [7] were used to calculate UO 2 thermal conductivity. All calculations were performed with the scalable parallel short-range MD code [32] and closely follow the study by Watanabe et al . [8] A constant heat flow was imposed in a rectangular cuboid simulation cell by allowing thermal energy to transmit from a hot plate to a cold plate separated by half of the simulation cell length. The thickness of the hot and cold plates was 5.463 Å, that is, one UO 2 unit cell. The heat flow was set to 0.05 k B T / A ( k B is the Boltzmann constant and T is the temperature) per time step, where A is the cross section area of the simulation cell. Periodic boundary conditions were applied to the simulation cell. The size of the time step was 1.0 fs in all simulations. To equilibrate the thermal and strain properties of the system, each simulation was initiated by performing constant temperature and pressure simulations for 12.5 ps. The equilibration time after setting up the heat flow was 500 ps, and 500–1,000 ps were used as the data acquisition time. The temperature gradient resulting from the heat flux was monitored and averaged over the acquisition time to obtain the thermal conductivity via Fourier’s law, , where J z is the imposed heat flux, z represents the crystallographic direction of the temperature gradient and κ z is the effective conductivity in this direction. The inter-atomic forces between uranium and oxygen atoms were described by the short-range potential according to the study by Basak et al . [31] , and the long-range electrostatic interactions were calculated by the Wolf summation method [33] . The length of simulation cells ranged from 16 to 60 nm for the simulations along the <100> <110> and <111> crystallographic directions. These relatively short cells suffer from significant phonon scattering from the hot and cold plates, especially at low temperature. This is an artifact of the simulation setup, but the small cells are nevertheless useful for establishing physical trends and the results for infinite cell length can be obtained by extrapolation of to (refs 7 , 8 ), where c is a constant related to scattering by the hot and cold plates, L z is the length of the simulation cell and κ ∞ is the thermal conductivity for a simulation cell of infinite length. Due to the non-linear effects in the <100> direction originating from the ellipsoidal character of the projected oxygen trajectory shown in Fig. 1b , the following quadratic ( ) relation was also used for extrapolation , where c 1 and c 2 are constants. As for the linear model, c 1 captures the scattering from the hot and cold plates, while c 2 is related to the UO 2 lattice properties, which includes the ellipsoidal behavior of the oxygen trajectory in Fig. 1b . In the directions perpendicular to the thermal current, the simulation cells have lengths ranging from 3.7 to 4.0 nm. The dependence of the computed thermal conductivity on cross-sectional area has been shown to be weak [34] . However, for UO 2 , the dimensions of the simulation cell impact the ellipsoidal character of the projected oxygen trajectory illustrated in Fig. 1b . If the simulation in Fig. 1b is carried out in a cubic cell, the shape of the corresponding trajectory is spherical, which is expected for perfectly cubic or isotropic materials. This implies that the cuboid simulation cell slightly, but significantly, perturbs the UO 2 lattice properties, which is likely related to the soft C 44 elastic constant [28] . Ultimately, this perturbation results in anisotropic thermal conductivity. Ballistic phonon transport, which occurs if scattering of phonons in the simulation cell is minimal, is another possible explanation for the anisotropy. This is because under ballistic conditions, thermal conductivity is a fourth rank tensor related to the elastic stiffness tensor and anisotropic thermal conductivity could arise in cubic materials [2] , [3] . In the MD simulations, ballistic transport is intertwined with the dependence of thermal conductivity on the simulation cell length and scattering by the hot and cold plates. The extrapolation scheme should eliminate ballistic contributions, however it cannot be conclusively ruled out based on the present simulations. The results obtained from the scalable parallel short-range MD code in this study were also confirmed using the LAMMPS MD code [35] . Thermal conductivity measurements The depleted UO 2 single crystals used for the thermal conductivity measurements were obtained by the Los Alamos Scientific Laboratory (LASL, now Los Alamos National Laboratory—LANL) from the Battelle Northwest Laboratory in 1969. Samples were prepared by fusing depleted PWR-grade UO 2 powder in an arc furnace and large crystals were harvested from the bulk [36] . Before delivery to LASL, crystals were annealed in moist hydrogen to remove inclusions and assure stoichiometry. We performed thermal gravimetric analysis on the samples studied and the results confirmed the original assertion of stoichiometry to be <2.001 (original coulometric titration in 1969 resulted in a stoichiometry of 2.0006). Regarding chemical purity, analysis performed at the time of original synthesis confirmed high purity samples (>99.9688%). By emission spectrographic analysis Ag, B, Fe, Sn and so on were below 200 ppm total, C below 50 ppm, Cl less than 10 ppm and F less than 2 ppm. The total nitrogen content was found to be 50 ppm as determined by Kjeldahl analysis. The isotopic purity of the samples was 238 U >99.78% (the balance is 235 U). Optical microscopy showed the samples to be free of macroscopic defects (cracks and so on). Oriented rectangular cuboids were prepared from a large single crystal, see Supplementary Fig. 1 for an example of the crystal bars, and orientations were verified by standard Laue back-reflection X-ray technique. As an example Supplementary Fig. 2 shows a typical Laue diffraction pattern for <111> samples. The character of the pattern highlights the high quality of the crystal. The misalignment is estimated to be <0.5 degrees for all samples. In addition, we prepared a <110> sample that was misaligned by 8 degrees. The thermal conductivity of the second <110> crystal was almost identical to the first sample. The close agreement between the two <110> crystals also confirms that the original single crystal was homogeneous, and thus our results of anisotropic thermal conductivity cannot be explained by variations in the UO 2 crystal properties between the oriented samples. This is further evidenced by the fact that the difference in the thermal conductivities between the <110> <111> and <100> samples approaches zero at the Néel temperature. X-ray diffraction was also performed on all of the single crystal samples, which confirmed the fluorite structure and lattice parameters consistent with literature data. The UO 2 thermal conductivity measurements were performed in a Physical Property Measurement System-9 from Quantum Design equipped with a 9 T superconducting magnet and using samples with typical dimensions of ~1 × 1 × 7 mm. Both four-terminal and two-terminal probe lead configurations were used to measure thermal conductivity. A silver-filled H20E epoxy was used to connect the sample to the leads, which are gold-coated copper. We used the continuous mode (0.1 Kmin −1 ) in the temperature range 4–300 K. To gain down the bridge, it is important to use 40 mV as the upper power limit because the resistivity of the sample is in the kOhm regime (at room temperature). According the Quantum Design handbook the typical accuracy, taking into account radiation losses, of thermal conductivity measurements using a TTO option is ±5%. However, since our measurements are performed on the same material, the relative accuracy between the oriented samples is much higher. To ensure that the sample mounting, for example, the leads attached to the ends of the UO 2 samples, did not bias the results, we demounted the <100> and <110> samples, annealed them in dry Ar-6%H 2 gas at 850°C for 18 hours to ensure sample stoichiometry, remounted the sample and repeated the thermal conductivity measurements, which reproduced the original results. The variation was well within the uncertainty range of the methodology, which confirms the validity of the anisotropic thermal conductivity. The second measurement series used two instead of four wire terminals. The <110> and <111> results agree with earlier single crystal measurements [2] and they are thus deemed to be accurate. We reiterate that any defects differentiating the <110> <111> and <100> samples would result in a constant shift in the thermal conductivities, which is not observed in our measurements, see Fig. 2 . A final argument against sample defects or concerns about the sample mounting is obtained by comparing the anisotropy at, for example, the maximum of the low temperature thermal conductivity peak with the anisotropy for the same magnitude of the conductivity at the second peak. The anisotropy is not the same, which should be the case if defects or inaccurate sample mounting were responsible for the measured anisotropy. From this we conclude that the anisotropic thermal conductivity cannot be explained by simple defects or measurement uncertainties. The Callaway model Above T N the measured thermal conductivities were analyzed in terms of the Callaway model [21] , which assumes a Debye phonon spectrum and expresses thermal conductivity as: where ν is the mean velocity of sound, τ p stands for the phonon relaxation time, x = ħω / k B T , ω is the phonon frequency, while ħ , Θ D and k B are the reduced Planck constant, the Debye temperature and the Boltzmann constant, respectively. The mean sound velocity was taken as ν =3,171 m s −1 for UO 2 , which was calculated from ( Θ D =395 K [37] ), where n is the number of atoms per unit volume. The relaxation time may be accounted for by considering possible scattering mechanisms for heat transport. This typically includes point defect scattering ( D ), boundary scattering ( B ), Umklapp processes ( U ) and spin scattering ( S ), , where the particular inverse relaxation times are given by the following expressions ( D , B and U are constants fitted to thermal conductivity data): The spin scattering term [22] is an extension to the standard Callaway model, which is required for paramagnetic UO 2 . In the expression for , ω S , i is the resonance frequency, C i the phonon-spin coupling constant and F i ( T ) contains information about the two-level system. We included two levels in our model ( i =1,2). Both the resonance frequencies and coupling constants were treated as free parameters. The b parameter in the Umklapp expression is here treated as a fitting parameter, but it may also be set to a constant ( b =2). To have a realistic starting point for the free parameters in the UO 2 model, we used the Callaway model parameters derived for ThO 2 from the data reported in ref. 14 . The mean sound velocity for ThO 2 was calculated to be 2,129 m s −1 for Θ D =259 K [38] . The ThO 2 results are listed in Supplementary Table 1 and compared with the experimental data in Supplementary Fig. 3 . For UO 2 , we first fit the <110> data by a Callaway model that does not include the phonon-spin scattering contribution (UO 2 <110> B in Supplementary Table 1 and Supplementary Fig. 3 ). The results are somewhat unusual on initial inspection; in particular the mean free path for boundary scattering is extremely low (7.3 nm). The boundary term is many orders of magnitude smaller than the dimensions of the sample. This can be explained by phonon-spin scattering, which is not explicitly included in the standard Callaway model, but rather captured by the boundary term. Note that the boundary scattering term for ThO 2 gives a mean free path of 8.0 μm, which is more than three orders of magnitude larger than for UO 2 (7.3 nm), as explained by the lack of phonon-spin scattering in ThO 2 . The fact that the defect scattering terms are similar between UO 2 and ThO 2 , see Supplementary Table 1 , indicates that isotopic scattering is not responsible for the difference in thermal conductivity. Although the UO 2 samples are not completely isotopically pure (99.78%) and the ThO 2 samples are, the high mass of U atoms means that isotope scattering is small in comparison to phonon-spin scattering. Even though the quality of the UO 2 fits obtained from the standard Callaway model is good, the physical insights that can be gained from these results are limited. In the next step, we added the spin scattering terms to the Callaway model, which we label the extended Callaway model, and fitted the UO 2 <110> thermal conductivity data, see Supplementary Table 1 and Fig. 3 , starting from the ThO 2 parameters. The reduced UO 2 thermal conductivity compared with ThO 2 is captured by the spin scattering terms and a decrease in the defect scattering length. The boundary scattering term remains similar to the ThO 2 case. The two resonance frequencies essentially overlap for the <110> fit. The <111> and <100> UO 2 thermal conductivity data was then fitted by only allowing the spin scattering terms to change, keeping all other parameters fixed at the <110> values, see Supplementary Table 1 and Fig. 3 . The quality of the <111> fit is excellent and for <100> it is also good, even though not perfect. For <100> a better fit is easily obtained by allowing the Umklapp parameters to change, see Supplementary Table 1 and Fig. 3 . Compared with the extended Callaway model for the <110> conductivity, the <111> and <100> anisotropies are accommodated by shifting and splitting the spin resonance frequencies or energies and slightly modifying the phonon-spin coupling terms. As discussed in Results, we propose that these changes are induced by the temperature gradient applied in the thermal conductivity experiments. How to cite this article: Gofryk, K. et al . Anisotropic thermal conductivity in uranium dioxide. Nat. Commun. 5:4551 doi: 10.1038/ncomms5551 (2014).